Drug screening inScn1azebrafish mutant identifies clemizole as a potential Dravet syndrome treatment Dravet syndrome is a catastrophic pediatric epilepsy with severe intellectual disability, impaired social development and persistent drug-resistant seizures. One of its primary monogenic causes are mutations in Na v 1.1 ( SCN1A ), a voltage-gated sodium channel. Here we characterize zebrafish Na v 1.1 ( scn1Lab ) mutants originally identified in a chemical mutagenesis screen. Mutants exhibit spontaneous abnormal electrographic activity, hyperactivity and convulsive behaviours. Although scn1Lab expression is reduced, microarray analysis is remarkable for the small fraction of differentially expressed genes (~3%) and lack of compensatory expression changes in other scn subunits. Ketogenic diet, diazepam, valproate, potassium bromide and stiripentol attenuate mutant seizure activity; seven other antiepileptic drugs have no effect. A phenotype-based screen of 320 compounds identifies a US Food and Drug Administration-approved compound (clemizole) that inhibits convulsive behaviours and electrographic seizures. This approach represents a new direction in modelling pediatric epilepsy and could be used to identify novel therapeutics for any monogenic epilepsy disorder. Epilepsy can be acquired as a result of an insult to the brain or genetic mutation. Among the genetic epilepsies, more than 650 variants have been identified in the SCN1A gene [1] , [2] . Missense or frame-shift mutations in this gene are associated with generalized epilepsy with febrile seizures plus [3] as well as a more severe disorder known as Dravet syndrome (DS). Children with DS initially exhibit normal development but often experience febrile seizure episodes within the first year of life, with eventual progression to severe spontaneous recurrent seizures, intellectual disability, ataxia and psychomotor dysfunction. Seizures are inadequately managed using available antiepileptic drugs (AEDs) and these children are poor candidates for neurosurgical resection [4] . In mammalian brain, there are four main subtypes of voltage-gated sodium channel α-subunits: Na V 1.1, Na V 1.2, Na V 1.3 and Na V 1.6, encoded for by the genes SCN1A , SCN2A , SCN3A and SCN8A , respectively. Opening of these channels produces a sodium conductance and rapid cell membrane depolarization, for example, features integral to action potential initiation [5] . In mice, Na v 1.1 is widely expressed in the central nervous system (CNS), including the axon initial segment of parvalbumin-positive hippocampal interneurons and excitatory principal cells [6] , [7] . Heterozygous deletion of Na v 1.1 in mice leads to a reduction in the firing capability of acutely dissociated fast-spiking interneurons [8] . Mice with global or interneuron-specific heterozygous deletion of Na v 1.1 exhibit temperature-induced and spontaneous seizures, mild ataxia, autism-like behaviours and premature death [8] , [9] , [10] . Knock-in mouse carrying a premature stop codon in domain III of the Na v 1.1 channel also exhibit a decrement in spike amplitude during prolonged interneuron firing and increased sensitivity to temperature-induced seizures [11] . Generation and characterization of valid animal models is critical to efforts to understand the pathophysiology of DS, and to aid in the identification of novel therapies. Although considerable attention has focused on modelling SCN1A mutations in mice, these animals have proven to be difficult to breed, and epilepsy phenotypes are strongly influenced by the background strain genetics. Induced pluripotent stem cells can be generated from DS patients, but individual neurons do not recapitulate the network environment necessary for in-vivo seizure generation. Danio rerio (zebrafish), a simple vertebrate species, provide an alternative model system with significant advantages for genetic manipulation, cost-efficient breeding and in-vivo drug discovery [12] , [13] , [14] . Ideally, an animal model should be based on a known genetic cause of the disease ( SCN1A mutation), accurately recapitulate key features of the disease (epilepsy), and respond, or not, to therapies commonly used in patients with the disease (pharmacological validation). If successful, such a model could inform our understanding of the disease process and catalyse explorations towards new therapies. In zebrafish, the voltage-gated sodium channel family consists of four sets of duplicated genes: scn1Laa and scn1Lab , scn4aa and scn4ab , scn5Laa and scn5Lab , and scn8aa and scn8ab (ref. 15 ). The zebrafish scn1Lab gene shares a 77% identity with human SCN1A and is expressed in the CNS. A homozygous zebrafish mutant for this gene (originally termed didy s552 ) was discovered in a chemical mutagenesis screen using the optokinetic response as an assay [16] . These types of screens are based on inducing random point mutations using the alkylating agent N- ethyl -N- nitrosourea; the resulting mutations are typically loss-of-function and recessive. Although this is a homozygous mutation, scn1Lab zebrafish mutants are relevant for the autosomal dominant human DS given the genome duplication in zebrafish and the presence of an additional Na v 1.1 homologue ( scn1Laa ). In this paper, we characterized scn1Lab mutants at the molecular and behavioural level, demonstrated that mutants exhibit spontaneous drug-resistant seizures and then used them in a novel high-throughput screening programme to identify compounds that ameliorate the epilepsy phenotype. A phenotype-based screen identified clemizole, an US Food and Drug Administration (FDA)-approved compound, as an effective inhibitor of spontaneous convulsive behaviours and electrographic seizures in these mutants. Developmental scn1Lab expression and characterization Zebrafish with a mutation in domain III of a voltage-gated sodium channel were identified by Dr Herwig Baier during a chemical mutagenesis screen [16] . We backcrossed original scn1Lab mutants onto the Tupfel long background for seven to ten generations and confirmed a methionine (M) to arginine (R) mutation in our colony ( Fig. 1a ). Reverse-transcriptase and quantitative (q) PCR revealed a decrease in mRNA expression for scn1Lab in mutant larvae at 3, 5 and 7 days post fertilization (dpf; Fig. 1b ); antibodies recognizing this protein in zebrafish are not available. As expected [15] , scn1Lab is prominently expressed during early stages of larval development ( Fig. 1b ) and specifically in the CNS at 3 dpf ( Fig. 1d,e ). Whole-mount in situ hybridization revealed diffuse but prominent expression in the brain regions corresponding to the forebrain (telencephalon), optic tectum and cerebellum. A similar expression pattern was observed for scn1Laa at 3 dpf. At 5 and 7 dpf, CNS expression remained prominent and faint scn1Lab signal was also noted in the heart ( Fig. 1d ). Relative expression of scn8aa or scn8ab (Na v 1.6), for example, a subunit thought to act as a genetic modifier of DS [17] , failed to reveal a significant difference in the expression between mutants and sibling controls at 5 dpf ( Fig. 1c ). Similarly, microarray analysis at 5 dpf also failed to detect a compensatory change in the mRNA expression of 13 different zebrafish scn subunits ( Table I ), including the other homologue ( scn1Laa ). These results demonstrate a selective defect in a zebrafish Na v 1.1 gene expressed in the CNS during early development. 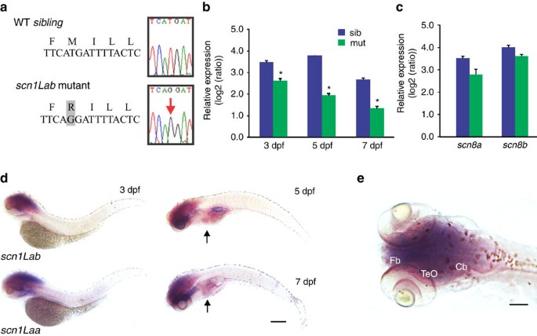Figure 1: Molecular characterization ofscn1Labzebrafish mutants. (a) Sequencing confirmed a T–G mutation inscn1Labmutant complementary DNA. (b) Verification of reduced expression inscn1Labmutants compared with sibling controls (Sib Ctrl) at 3, 5 and 7 dpf using qPCR. Data presented as mean±s.e.m.; *significance taken asP<0.05 Student’st-test. Data were normalized to the internal reference geneβ-actin. Values represent averages from five independent biological samples (one sample=ten pooled larvae) for each of the three developmental stages. Data presented as mean±s.e.m.; *significance taken asP<0.05 Student’st-test. (c) Relative expression ofscn8aaandscn8abin Nav1.1 mutants (n=5) and sibling controls (n=5) at 5 dpf. Data presented as inb. (d) Whole-mountin situhybridization forscn1Labin larval zebrafish at 3, 5 and 7 dpf. Wild-type larvae are shown in lateral views; expression is shown in dark purple.Scn1Laaexpression at 3 dpf is shown for comparison. Heart indicated by arrowheads in 5 and 7 dpf panels. (e) Dorsal view ofscb1Laaexpression at 3 dpf; note the prominent expression in regions corresponding to the larval zebrafish CNS. Cb, cerebellum; Tel, telencephalon; TeO, optic tectum; Scale bars, 0.35 mm ind, 0.2 mm ine. Figure 1: Molecular characterization of scn1Lab zebrafish mutants. ( a ) Sequencing confirmed a T–G mutation in scn1Lab mutant complementary DNA. ( b ) Verification of reduced expression in scn1Lab mutants compared with sibling controls (Sib Ctrl) at 3, 5 and 7 dpf using qPCR. Data presented as mean±s.e.m. ; *significance taken as P <0.05 Student’s t -test. Data were normalized to the internal reference gene β-actin . Values represent averages from five independent biological samples (one sample=ten pooled larvae) for each of the three developmental stages. Data presented as mean±s.e.m. ; *significance taken as P <0.05 Student’s t -test. ( c ) Relative expression of scn8aa and scn8ab in Na v 1.1 mutants ( n =5) and sibling controls ( n =5) at 5 dpf. Data presented as in b . ( d ) Whole-mount in situ hybridization for scn1Lab in larval zebrafish at 3, 5 and 7 dpf. Wild-type larvae are shown in lateral views; expression is shown in dark purple. Scn1Laa expression at 3 dpf is shown for comparison. Heart indicated by arrowheads in 5 and 7 dpf panels. ( e ) Dorsal view of scb1Laa expression at 3 dpf; note the prominent expression in regions corresponding to the larval zebrafish CNS. Cb, cerebellum; Tel, telencephalon; TeO, optic tectum; Scale bars, 0.35 mm in d , 0.2 mm in e . Full size image Table 1 scn channel subunit expression on microarray. Full size table Large-scale transcriptomic analysis of scn1Lab mutants Although inherited disorders of voltage-gated ion channels are recognized as an aetiology of epilepsy, investigation of transcriptional changes has not been reported for any epilepsy-related channelopathy. To detect differences in gene expression in an unbiased manner, we used an Agilent Danio rerio chip covering ~44,000 probes ( Fig. 2a,b ). Hierarchical clustering analyses showed that ~2.5% (1,099) of these probes (see Supplementary Data 1 ) were differentially expressed between mutants and sibling controls at 5 dpf ( P ≤0.01, Student’s t -test; 674 upregulated and 425 downregulated); 405 were assigned to an ‘unknown function’ category. A list of 30 down- and upregulated known genes showing the greatest differences in expression is shown in Fig. 2c . Surprisingly, these differences were modest as 90% (990/1,099) of the identified genes exhibited fold-changes between 0.8 and 2.0. Similar to microarray analysis of Mecp2 single-gene mutant mice [18] , many of the genes identified had no obvious CNS-related function and/or expression. The two largest fold-changed genes, somatolactin β , and a Na, K-ATPase, have expression primarily restricted to the pituitary ( smtlb ) [19] or the ear, intestinal bulb and pronephric duct ( atp1a1a.5 ) [20] . Probes for several genes related to apoptosis ( casp8 , casp8b and casp3b ) did not reveal any statistically significant changes in the microarray studies. Of the genes with altered expression in scn1Lab mutants, six were previously implicated in neurological disorders, for example, pcdh19 (infantile epileptic encephalopathy), cyfip1 and fxr2 (Fragile X syndrome), ocrl (Lowe syndrome), ubap2l (Parkinson’s disease) and oca2 (Angelman syndrome). Microarray-based gene expression measurements were verified for 14 randomly selected genes using qPCR ( Fig. 3a ). Biological functions were assigned to all genes using gene ontology annotations, and the 482 genes showing at least a 1.5-fold change in expression and a P value <0.01 were categorized further ( Fig. 3c ). Calcium ion binding genes include annexinA1c , A1b and 2a , spectrin α2 , neurexin 2a , calsyntenin 1 and parvalbumin 3 . Significant changes in a gap junction channel ( cx43 ), a gene involved in clustering of voltage-gated sodium channels at the axon initial segment ( spna2 ) and the ubiquitin domain of a GABA receptor ( map1lc3b ) were also noted. Three additional genes not found on the microarray were chosen for qPCR analysis ( Fig. 3b ): hcn1 , a gene shown to be correlated with SCN1A using data mining (Starnet2; http://vanburenlab.medicine.tamhsc.edu/starnet2.shtml ) and downregulated in several seizure models [21] was significantly reduced in scn1Lab mutants compared with that in sibling control ( P <0.05, two-tailed Student’s t -test). However, genes involved in synaptogenesis related to the formation of recurrent excitatory synapses and epilepsy [22] , [23] , for example, homer and bdnf , were unchanged. 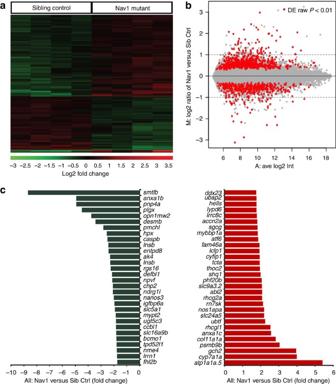Figure 2: Microarray analysis ofscn1Labzebrafish mutants. (a) Heat maps depicting the expression of genes differentially expressed betweenscn1Labmutant and sibling control (Sib Ctrl) larvae at 5 dpf. Rows represent individual genes. Columns represent different larvae. Genes that are highly expressed inscn1Labmutants relative to controls are shown in red. (b) MA plot of normalized microarray data for all 44,000 genes. The log-ratio M and the mean fluorescence intensity A were calculated as the averages for all replicates. (c) A list of the top 30 genes showing the greatest differences (upregulated genes are shown in red and downregulated genes are shown in blue) in expression betweenscn1Labmutants and Sib Ctrls. Figure 2: Microarray analysis of scn1Lab zebrafish mutants. ( a ) Heat maps depicting the expression of genes differentially expressed between scn1Lab mutant and sibling control (Sib Ctrl) larvae at 5 dpf. Rows represent individual genes. Columns represent different larvae. Genes that are highly expressed in scn1Lab mutants relative to controls are shown in red. ( b ) MA plot of normalized microarray data for all 44,000 genes. The log-ratio M and the mean fluorescence intensity A were calculated as the averages for all replicates. ( c ) A list of the top 30 genes showing the greatest differences (upregulated genes are shown in red and downregulated genes are shown in blue) in expression between scn1Lab mutants and Sib Ctrls. 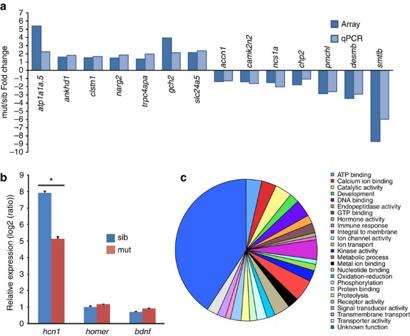Figure 3: Quantitative reverse-transcriptase PCR analysis ofscn1Labzebrafish mutants. (a) Comparison of the gene expression fold-changes obtained by microarray analysis (array) and real-time qPCR analysis. Theyaxis represents the average fold change in gene expression of each gene from zebrafish at 5 dpf. Thexaxis represents different genes. (b) qPCR analysis of three genes involved in epileptogenesis. The relative gene expression is presented as log2ratios to the least abundant transcript (log2ΔΔct). Data were normalized to the internal reference geneβ-actin. Values represent averages from five independent biological samples (one sample=ten pooled larvae). Bars indicate s.e.m.; *P<0.05 Student’st-test. (c) Gene ontology classification of differentially expressed genes detected inscn1Labmutants at 5 dpf (P<0.05, ANOVA one-way and fold-changes >1.5). Biological processes representing at least five gene annotations in at least one category are displayed. Full size image Figure 3: Quantitative reverse-transcriptase PCR analysis of scn1Lab zebrafish mutants. ( a ) Comparison of the gene expression fold-changes obtained by microarray analysis (array) and real-time qPCR analysis. The y axis represents the average fold change in gene expression of each gene from zebrafish at 5 dpf. The x axis represents different genes. ( b ) qPCR analysis of three genes involved in epileptogenesis. The relative gene expression is presented as log 2 ratios to the least abundant transcript (log 2 ΔΔct). Data were normalized to the internal reference gene β-actin . Values represent averages from five independent biological samples (one sample=ten pooled larvae). Bars indicate s.e.m. ; * P <0.05 Student’s t -test. ( c ) Gene ontology classification of differentially expressed genes detected in scn1Lab mutants at 5 dpf ( P <0.05, ANOVA one-way and fold-changes >1.5). Biological processes representing at least five gene annotations in at least one category are displayed. Full size image Spontaneous seizures in scn1Lab mutant zebrafish Next, we monitored scn1Lab mutants for evidence of spontaneous electrographic seizures starting at 3 dpf, for example, the first larval stage at which epileptiform discharge can be detected [24] , [25] , [26] , [27] , [28] . Mutant larvae were identified by their ‘black’ appearance ( Fig. 4a ), which is indicative of a defect in pigment aggregation and die prematurely between 10 and 12 dpf, as reported previously [15] . The forebrain extracellular field recordings from paralysed and agar-immobilized scn1Lab mutants were marked by frequent brief interictal-like bursts and large-amplitude, long-duration, ictal-like events starting at 3 dpf ( n =4) and progressively becoming more prominent between 4 and 7 dpf ( n =132; Fig. 2c ). These events were confirmed in 100% of mutants at 3 dpf, 100% at 4 dpf, 97% at 5 dpf, 98% at 6 dpf and 100% at 7 dpf. Temporal expansions of seizure activity and comparisons with single action potential and twitch artefact recordings are shown in Supplementary Fig. S1 . Abnormal electrical events were never observed in age-matched sibling controls at any developmental stage ( n =36). Hyperthermia-induced seizures [26] could be evoked in 5 dpf scn1Lab mutants and controls at apparently similar temperature thresholds (mutant: 26.9±0.5 °C; n =14; control: 25.9±0.5 °C; n =14; p =0.164, Student’s t -test). However, these measurements were complicated, in mutants, by simultaneous occurrence of high-frequency, spontaneous epileptiform discharges. Mutants had elevated levels of swim activity and exhibited unprovoked seizure-like behaviour consisting of whole-body convulsions and rapid undirected movement starting at 4 dpf ( n =36). A representative locomotion tracking plot of a scn1Lab mutant showing hyperactivity and convulsive behaviour is shown in Fig. 4b . This behaviour is similar to that classified as a Stage III seizure in larvae exposed to pentylenetetrazole [27] . Seizure behaviours were never observed in controls at any stage of development ( n =36). In pools of mutant and sibling control larvae, scn1Lab mutants stay close to the sides of the petri dish, which is considered a form of thigmotaxis in fish [29] . These results reveal a striking epilepsy phenotype in scn1Lab mutant zebrafish. 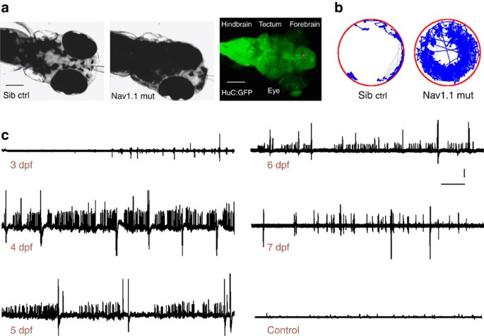Figure 4: Spontaneous seizures inscn1Labzebrafish mutants. (a) Immobilized and agar-embedded zebrafish larvae are shown. Images were obtained using a × 4 objective and × 2 magnifier on an Olympus upright microscope during forebrain electrophysiological recordings in sibling control (Sib Ctrl) (a, left) andscn1Labmutant (a, middle) larvae at 5 dpf. Note the dark pigmentation for mutants. Recording electrodes can be seen ina(left and middle) and the approximate site of the recording electrode tip in the forebrain (red circle) is shown using a representative HuC:GFP-labelled larvae ina(right). Scale bar, 100 μm. (b) Sample locomotion tracking plot for Sib ctrl (b, left) andscn1Labmutant (b, right) larvae at 5 dpf. (c) Representative 10 min recording epochs obtained in the forebrain of paralysed, immobilized and agar-embeddedscn1Labmutant larvae between 3 and 7 dpf. Note the presence of small and large amplitude spontaneous burst discharge; additional temporal expansions of seizure activity are shown inSupplementary Fig. S1. A representative recording, under identical recording conditions, from an Sin Ctrl larvae at 5 dpf is also shown. Scale bar, 2 mV; 30 s. Figure 4: Spontaneous seizures in scn1Lab zebrafish mutants. ( a ) Immobilized and agar-embedded zebrafish larvae are shown. Images were obtained using a × 4 objective and × 2 magnifier on an Olympus upright microscope during forebrain electrophysiological recordings in sibling control (Sib Ctrl) ( a , left) and scn1Lab mutant ( a , middle) larvae at 5 dpf. Note the dark pigmentation for mutants. Recording electrodes can be seen in a (left and middle) and the approximate site of the recording electrode tip in the forebrain (red circle) is shown using a representative HuC:GFP-labelled larvae in a (right). Scale bar, 100 μm. ( b ) Sample locomotion tracking plot for Sib ctrl ( b , left) and scn1Lab mutant ( b , right) larvae at 5 dpf. ( c ) Representative 10 min recording epochs obtained in the forebrain of paralysed, immobilized and agar-embedded scn1Lab mutant larvae between 3 and 7 dpf. Note the presence of small and large amplitude spontaneous burst discharge; additional temporal expansions of seizure activity are shown in Supplementary Fig. S1 . A representative recording, under identical recording conditions, from an Sin Ctrl larvae at 5 dpf is also shown. Scale bar, 2 mV; 30 s. Full size image Pharmacological evaluation of scn1Lab mutant zebrafish Seizures associated with SCN1A mutations are poorly responsive to most AEDs. To evaluate pharmaco-sensitivity, we recorded spontaneous electrographic seizures in agar-embedded scn1Lab mutants (5–6 dpf) under baseline conditions, and again after application of a commercially available AED. All drugs were bath applied at a concentration of 1 mM; seven fish were tested for each drug. Epileptiform event frequency (including interictal- and ictal-like discharges) and the fractional time spent seizing in scn1Lab mutants were reduced by valproate, diazepam, potassium bromide and stiripentol ( Fig. 5a,b,d ). Burst durations were not significantly changed for any of these drug exposures ( Fig. 5c ). As expected, most AEDs had no effect and epileptiform activity became more frequent following exposure to carbamazepine (in two out of seven fish), ethosuximide (four out of seven fish) or vigabatrin (six of seven fish). As DS children often respond to the ketogenic diet (KD) [30] , we exposed a separate clutch of scn1Lab mutants, siblings and wild-type (WT) controls to a form of the diet [31] for 48 h starting at 4 dpf. Locomotion tracking data on KD-exposed larvae at 6 dpf confirm a reduction in seizure-like behaviour to control levels in seven out of ten mutants ( Fig. 5e ; mean velocity, treated mutants=0.43±0.09 mm s −1 , n =16; untreated mutants=0.81±0.05 mm s −1 , n =28; P <0.05, Kruskal–Wallis analysis of variance (ANOVA) on Ranks with a Dunn’s pairwise multiple comparison). No significant differences in swim behaviour were noted in sibling controls treated with the KD (mean velocity=0.63±0.05 mm s −1 , n =20) compared with untreated WT larvae at 6 dpf (mean velocity=0.62±0.07 mm s −1 ; n =20). Acute exposure (20 min) to the diet had no effect on mutant seizure behaviour in the locomotion assay ( n =14; change in mean velocity <34%). Subsequent forebrain field recordings obtained from the same zebrafish used in the locomotion assay ( Fig. 5f , top trace) confirmed the occurrence of spontaneous epileptiform discharge for embryo media exposed scn1Lab mutants and a suppression of burst activity in mutants exposed to the KD for 48 h ( Fig. 5f , bottom trace). These results demonstrate that the pharmacological profile for scn1Lab mutants resembles that seen in children with DS. 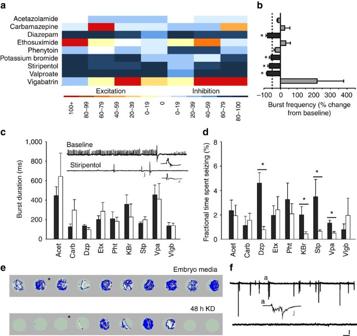Figure 5: Pharmacological validation ofscn1Labzebrafish mutants. (a) Heat map showing the response to nine different AEDs. Each column represents the per cent change in burst frequency (baseline—drug/baseline × 100) for one individual zebrafish mutant. Drugs that inhibit seizure events are shown in dark blue. All drugs were tested at a concentration of 1 mM. Note in some trials, carbamazepine and vigabatrin increased burst frequency over the initial baseline levels. (b) Plot of the mean change in burst frequency and s.e. for the data shown in the heat map. Pairedt-test or Wilcoxon signed-rank sum test for data that failed the normality test showed significance as follows: diazepam (P=0.002;n=7), potassium bromide (P=0.016;n=7), stiripentol (P=0.024;n=7) and valproate (P=0.004;n=7). (c) Plot of the burst duration for all trials shown ina. Data are presented as the mean±s.e.m. for electrographic seizure events at baseline (black bars) and after drug exposure (white bars). Inset shows a representative 2-min recording during the stiripentol trial; scale bars, large trace 1 mV, 1 s; small trace 1 mV, 100 ms. (d) Plot of the fractional time spent seizing for all trials shown ina. Data are presented as the mean±s.e.m. for electrographic seizure events at baseline (black bars) and after drug exposure (white bars). Student’st-test or Mann–Whitney–Rank sum test for data that failed the normality test showed significance as follows: diazepam (P=0.001;n=7); potassium bromide (P=0.043;n=7); stiripentol (P=0.007;n=7) and valproate (P=0.007;n=7). (e) Locomotion tracking plots for ten individual mutant larvae raised in embryo media (top row) or the KD for 48 h. Plots show swim velocity and locomotion tracks with darker colours indicative of higher velocities; 10-min trials are shown. (f) Representative 10-min extracellular recording epochs from the same fish shown ine; representative examples are indicated by * in the locomotion plots. Scale bar, 1 mV, 30 s. Inset shows burst at higher temporal resolution (indicated by #); scale bar, 1 mV, 100 ms. Figure 5: Pharmacological validation of scn1Lab zebrafish mutants. ( a ) Heat map showing the response to nine different AEDs. Each column represents the per cent change in burst frequency (baseline—drug/baseline × 100) for one individual zebrafish mutant. Drugs that inhibit seizure events are shown in dark blue. All drugs were tested at a concentration of 1 mM. Note in some trials, carbamazepine and vigabatrin increased burst frequency over the initial baseline levels. ( b ) Plot of the mean change in burst frequency and s.e. for the data shown in the heat map. Paired t -test or Wilcoxon signed-rank sum test for data that failed the normality test showed significance as follows: diazepam ( P =0.002; n =7), potassium bromide ( P =0.016; n =7), stiripentol ( P =0.024; n =7) and valproate ( P =0.004; n =7). ( c ) Plot of the burst duration for all trials shown in a . Data are presented as the mean±s.e.m. for electrographic seizure events at baseline (black bars) and after drug exposure (white bars). Inset shows a representative 2-min recording during the stiripentol trial; scale bars, large trace 1 mV, 1 s; small trace 1 mV, 100 ms. ( d ) Plot of the fractional time spent seizing for all trials shown in a . Data are presented as the mean±s.e.m. for electrographic seizure events at baseline (black bars) and after drug exposure (white bars). Student’s t -test or Mann–Whitney–Rank sum test for data that failed the normality test showed significance as follows: diazepam ( P =0.001; n =7); potassium bromide ( P =0.043; n =7); stiripentol ( P =0.007; n =7) and valproate ( P =0.007; n =7). ( e ) Locomotion tracking plots for ten individual mutant larvae raised in embryo media (top row) or the KD for 48 h. Plots show swim velocity and locomotion tracks with darker colours indicative of higher velocities; 10-min trials are shown. ( f ) Representative 10-min extracellular recording epochs from the same fish shown in e ; representative examples are indicated by * in the locomotion plots. Scale bar, 1 mV, 30 s. Inset shows burst at higher temporal resolution (indicated by #); scale bar, 1 mV, 100 ms. Full size image High-throughput drug screening in scn1Lab mutants As the behavioural seizure activity is easily and rapidly monitored using a locomotion tracking format [24] , [25] , [27] , [28] , [32] , [33] , [34] , [35] , [36] ( Figs 4b and 5e ), we designed a relatively high-throughput phenotype-based strategy to screen chemical libraries for compounds that reduce mutant behaviour to Stage 0 (very little swim activity) or Stage I (increased, but non-convulsive, swim activity), for example, behaviour equivalent to that seen in normal WT controls. Automated measurement of larval activity was achieved using EthoVision tracking software (Noldus Information Technology) and a high-speed camera. Previous studies confirmed that high-velocity movement ≥20 mm s −1 correspond to paroxysmal seizure-like convulsions (Stage III) [35] , [36] . Using a 96-well format, we automatically tracked mutant swim activity at baseline, and then again after addition of a test compound (100 μl); each compound was tested on 6–12 individual larvae at 5 dpf. The change in mutant swim activity between two consecutive recording epochs in the embryo media was taken as baseline and is shown in Fig. 6a ( n =28). On the basis of an s.d. of 17.3 for baseline recordings associated simply with a solution exchange, we screened for compounds that inhibited movement (measured as a change in mean velocity) by ≥34%. To validate this approach, we first screened 11 AEDs and the KD using this assay. As expected from electrophysiological assays ( Fig. 5 ), diazepam, potassium bromide, stiripentol, valproate and a 48-h exposure to KD effectively inhibited seizure behaviour in the locomotion-based assay ( Fig. 6b ); ganaxolone, a neuroactive steroid related to allopregnalone, was also effective. Next, we screened test compounds at an initial concentration of 667 μM from a library that included the US FDA-approved and toxicology-tested drugs (the International Drug Collection; http://www.msdiscovery.com/spectrum.html ). Among the 320 compounds screened in vivo , 18 were found to significantly inhibit spontaneous seizures in scn1Lab mutants to levels comparable to Stage 0 or Stage I behaviour and/or reduce mean swim velocity (red circles in Fig. 6c ). These 18 compounds were then re-tested on a separate clutch of scn1Lab mutants at concentrations of 667, 67 and 6.7 μM. In the initial screen, 81 compounds were identified as lethal, that is, no visible heartbeat or movement in response to touch after a 30-min exposure (see Supplementary Table S1 ) and were re-evaluated at a dilution of 1:100; none of these advanced further. The drug library included a number of additional compounds with putative anticonvulsant properties (beclamide, aminohydroxybutyric acid and tiletamine) that were also ineffective in the 96-well locomotion assay at 667 μM. Fourteen of the re-tested compounds either failed to successfully inhibit seizure behaviour in a second clutch of scn1Lab mutants or only suppressed behaviour at the highest drug concentration. Next we selected 4 (out of 18) compounds that were effective in reducing seizure-induced swim activity and mean velocity at all 3 drug concentrations for further testing: zoxazolamine, clemizole HCl, clorgiline HCl and tolperisone HCl ( Fig. 6d ). Each of these compounds was evaluated a third time in the locomotion assay at a concentration of 100 μM, and subsequently monitored for forebrain electrographic activity. Clorgiline (a monoamine oxidase A inhibitor) and the muscle relaxants zoxazolamine [37] and tolperisone [38] were identified as ‘false positives’, because they reduced swim activity at this concentration, but when the same mutant was embedded in agar electrographic seizure events were still observed (see Fig. 6e ). Only one compound, clemizole (antihistamine and NS4B RNA binding inhibitor) [39] , [40] , was effective in suppressing spontaneous seizure activity in both assays ( Fig. 6d,e ). A comparison of electrophysiological burst characteristics for untreated ( n =3) and clemizole-treated ( n =7) scn1Lab mutants shown in Fig. 6e zebrafish indicates a statistically significant suppression of activity (untreated: burst frequency=1.5±0.3 bursts min −1 ; burst duration=926±414 ms; fractional time spent seizing=0.73±0.17%; versus clemizole: burst frequency=0.2±0.01 bursts min −1 ; burst duration=154±127 ms; fractional time spent seizing=0.03±0.02%; P =0.001 for all comparisons, Kruskal–Wallis ANOVA with a Dunn’s pairwise multiple comparison test). Clemizole had no significant effect on seizure behaviour in the locomotion assay at concentrations between 6.25 and 50 μM ( n =33). As an additional evaluation of the therapeutic potential for acute clemizole treatment, we also demonstrated that 100 μM clemizole was effective in reducing seizure behaviour in WT zebrafish exposed to 15 mM pentylenetetrazole ( Fig. 6d ; n =10), that is, a model of acute seizures based on GABA receptor antagonism. These results suggest that scn1Lab mutants can be used in a high-throughput screen to identify potential lead compounds for DS. 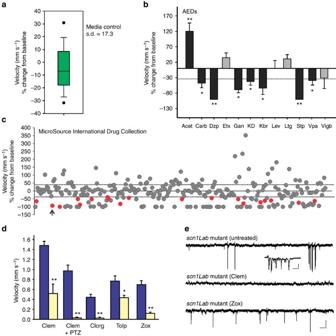Figure 6: Screen to identify drugs that rescuescn1Labmutant epilepsy phenotype. (a) Box plot of mean velocity (in mm s−1) for two consecutive recordings of mutant larvae in embryo media. The per cent change in velocity from baseline (recording 1) versus experimental (recording 2) is shown. The bottom and top of the box represent the 25th and 75th percentile, respectively. The horizontal line represents median value; vertical lines encompass the entire range of values. (b) Plot of the effect of AEDs on seizure behaviour inscn1Labmutants. Bars represent per cent change in mean velocity; 6–12 fish per experiment. Drugs tested at 1 mM; diazepam (Dzp;P<0.001), carbamazepine (Carb;P=0.024), ganaxolone (Gan;P=0.003), stiripentol (Stp;P=0.001), valproate (Vpa;P=0.026) and a 48-h KD (P=0.003) exposure reduced seizure activity, measured as a change in velocity, by more than the s.d. in control recordings (34%, dotted line). Acetazolamide (Acet;P<0.001) and ethosuximide (Etx;P=0.250) increased seizure behaviour; levetiracetam (Lev;P=0.243) and lamotrigine (Ltg;P=0.058) had no effect. (c) Plot for all 320 compounds tested. Coloured circles (red) represent positive hits; compounds that decreased the activity by 100% were generally toxic; 6–12 fish per trial. Arrowhead; first clemizole trial. (d) Plot of drug re-trials on separate mutant clutches; 100 μM per drug; ten fish per trial. Abbreviations: Clem, clemizole; Clem+PTZ, clemizole+15 mM PTZ; Clorg, clorgiline; Tolp, tolperisone; Zox, zoxazolamine. Effect of acute clemizole on PTZ-induced seizures shown for WT larvae. Bars represent mean±s.e.m. For panelsbandd: Student’s pairedt-test or Mann–Whitney–Rank sum test with significance set at *P=0.01 or **P<0.001. (e) Sample electrophysiology recordings fromscn1Labmutants exposed to clemizole in the locomotion assay (d) and then monitored using a forebrain recording (top trace; ictal-like burst shown in inset). Similar traces for an untreated mutant (middle) and mutant treated with zoxazolamine (bottom). Scale bars, large traces 0.5 mV, 10 s; inset 0.5 mV, 100 ms. Figure 6: Screen to identify drugs that rescue scn1Lab mutant epilepsy phenotype. ( a ) Box plot of mean velocity (in mm s −1 ) for two consecutive recordings of mutant larvae in embryo media. The per cent change in velocity from baseline (recording 1) versus experimental (recording 2) is shown. The bottom and top of the box represent the 25th and 75th percentile, respectively. The horizontal line represents median value; vertical lines encompass the entire range of values. ( b ) Plot of the effect of AEDs on seizure behaviour in scn1Lab mutants. Bars represent per cent change in mean velocity; 6–12 fish per experiment. Drugs tested at 1 mM; diazepam (Dzp; P <0.001), carbamazepine (Carb; P =0.024), ganaxolone (Gan; P =0.003), stiripentol (Stp; P =0.001), valproate (Vpa; P =0.026) and a 48-h KD ( P =0.003) exposure reduced seizure activity, measured as a change in velocity, by more than the s.d. in control recordings (34%, dotted line). Acetazolamide (Acet; P <0.001) and ethosuximide (Etx; P =0.250) increased seizure behaviour; levetiracetam (Lev; P =0.243) and lamotrigine (Ltg; P =0.058) had no effect. ( c ) Plot for all 320 compounds tested. Coloured circles (red) represent positive hits; compounds that decreased the activity by 100% were generally toxic; 6–12 fish per trial. Arrowhead; first clemizole trial. ( d ) Plot of drug re-trials on separate mutant clutches; 100 μM per drug; ten fish per trial. Abbreviations: Clem, clemizole; Clem+PTZ, clemizole+15 mM PTZ; Clorg, clorgiline; Tolp, tolperisone; Zox, zoxazolamine. Effect of acute clemizole on PTZ-induced seizures shown for WT larvae. Bars represent mean±s.e.m. For panels b and d : Student’s paired t -test or Mann–Whitney–Rank sum test with significance set at * P =0.01 or ** P <0.001. ( e ) Sample electrophysiology recordings from scn1Lab mutants exposed to clemizole in the locomotion assay ( d ) and then monitored using a forebrain recording (top trace; ictal-like burst shown in inset). Similar traces for an untreated mutant (middle) and mutant treated with zoxazolamine (bottom). Scale bars, large traces 0.5 mV, 10 s; inset 0.5 mV, 100 ms. Full size image The scn1Lab zebrafish mutant described here is the first simple vertebrate model of a sodium channel mutation that recapitulates features of DS, a catastrophic form of drug-resistant epilepsy in children. We have shown that these mutants exhibit hyperactivity, including convulsive behaviour, spontaneous electrographic seizures, shortened lifespan and a pharmacological profile similar to the human condition. Additional molecular analysis of scn1Lab mutants suggests the absence of gross changes in global gene expression and a lack of compensation, at the RNA level, by other voltage-gated Na + channel subunits. A two-stage phenotype-based drug screening strategy to identify lead compounds with the potential to ameliorate epilepsy phenotypes associated with SCN1A mutation identified one FDA-approved drug (clemizole). Electroencephalographic activity is typically normal in the first year of life for DS patients, with an evolution to abnormal paroxysmal and polyspike activity between 1 and 9 years of age. This age-dependent pattern was mimicked in the developing zebrafish larvae at ages where scn1a expression was significant. The forebrain extracellular recordings in very young larvae (3 dpf) appeared largely normal with the occasional small burst of polyspike activity. Frequent brief interictal-like activity with large amplitude polyspike burst discharges became more prominent as larvae aged. The architecture of these electrical events resembled those previously described in WT larvae exposed to pentylenetetrazole [27] , 4-aminopyridine [24] , linopirdine [28] or hyperthermia [26] . The appearance of electrographic seizure activity corresponds with hyperactivity, full-body convulsions with associated high-velocity swim activity and brief loss-of-posture in freely behaving mutants. These types of spontaneous behaviours are never observed in WT larvae and, again, resemble those previously observed only during exposure to convulsant drugs. These behaviours are an indirect indicator of seizure activity and could be used for rapid in-vivo evaluation of drug treatments and lethality in a multi-well format using automated locomotion tracking software [32] , [33] , [35] . We also show that seizures in scn1Lab zebrafish mutants are responsive to the KD and four AEDs (for example, valproate, benzodiazepine, potassium bromide and stiripentol) prescribed clinically for patients with DS [41] . Interestingly, electrographic seizure events in scn1Lab mutants remained unchanged (or perhaps worsened) in response to several commercially available AEDs. Although it is possible that drug concentrations higher than 1 mM could be required to abolish electrical events, these would be considered high and potentially non-selective concentrations. In drug trials using an acute pentylenetetrazole (PTZ)-induced seizure model in larval zebrafish [24] , [32] , [33] , [42] , AED concentrations of 1 mM and below were often sufficient for assessing antiepileptic activity. With a failure to respond to ten different AEDs, this model fits the clinical definition of drug-resistant epilepsy [43] . For nearly 40 years, the discovery and identification of new AEDs has almost entirely been based upon preclinical animal models of acquired or acute seizures in rodents [44] . This approach successfully identified drugs that block generalized tonic–clonic seizures in humans [45] but remains time-consuming, resource intensive, expensive and laborious. Although testing against PTZ or other types of acquired seizures in zebrafish larvae may be more efficient than similar assays in rodents [32] , [33] , [42] , they ultimately should identify the same classes of compounds. In contrast, here we describe an alternative screening strategy using a 96-well format for rapid automated behavioural monitoring followed by a sensitive electrophysiological assay of spontaneous electrographic seizure activity in a mutant fish mimicking a known human genetic disorder. Our in-vivo strategy simultaneously monitors lethality and is not limited to SCN1A , but could be applied to any monogenic epilepsy disorder. Indeed, this phenotype-based approach could form the basis of a genetically informed or ‘personalized’ approach to drug discovery. Although genetically modified mice mimicking known SCN1A mutations and exhibiting epilepsy have been developed, breeding can be complicated, background strain can modify seizure phenotypes and AEDs are rarely tested in these animals. For example, in Scn1a RX/+ mutant mice, stiripentol and clobazam were only evaluated for effects on hyperthermia-induced seizure thresholds [46] . Treatment of Scn1a +/− mutant mice with clonazepam, an allosteric modulator of GABA-A receptors, rescued some of the autistic-like behaviours but was not evaluated as an antiepileptic [43] . Where drug-resistant rodent epilepsy models have been described, such as the subgroup of WT rats selected from kindling or post-status epilepticus models [47] , they remain only poorly characterized and are not suitable to initial high-throughput stages of drug screening. In contrast, using a zebrafish scn1Lab mutant with greater than 75% sequence identity for a human sodium channel mutation, we completed a large-scale transcriptomic profiling of over 44,000 probes, demonstrated a developmental progression of scn1Lab channel expression and epileptic phenotypes, analysed the effects of available antiepileptic therapies and screened a 320-compound chemical library against spontaneous unprovoked seizures. Although this first proof-of-principle screen was accomplished at 1 fish per well, 6–12 fish per trial and 1 trial per week, the ease with which zebrafish could be scaled upward (especially in a commercial setting) to study 100s to 1,000s of larvae per week make this an attractive system for a rapid large-scale, first-stage in-vivo drug discovery programme. Simultaneous in-vivo evaluation of toxicity—one of the greatest sources of failure in moving lead compounds from the bench to the clinic—is a critical advantage of our approach over available organotypic hippocampal culture- or in silica -based screening strategies. Although any animal model drug discovery data should be treated cautiously, clemizole, a compound with H1 antagonist and NS4B RNA-inhibiting properties [39] , [40] , is an FDA-approved drug with a safe toxicology profile emerged from this screen and offers an exciting starting point for further research. For example, although it was recently recognized that antihistamines inhibit induced seizures in neonatal rats [48] , this may not be the mechanism of action here, as four other H1 antihistamines (pimethixene maleate, chloropyramine HCl, mebhydrolin napthalenesulphonate and iproheptine) failed to suppress convulsive behaviour in scn1Lab mutants. Furthermore, evidence suggests the potential for H1 antihistamines to adversely modify seizures in children [49] , indicating that a more detailed analysis will be required to identify a mechanism of action. Given that clemizole was also effective in a zebrafish version of the Metrazol test, it may be worthwhile to pursue additional preclinical testing in the NIH-sponsored Anticonvulsant Drug Development Program at the University of Utah. Most importantly, our studies suggest that in-vivo drug screening and experimental analysis of scn1Lab mutant zebrafish could prove extremely valuable to the understanding (and treatment) of DS. Animals Scn1Lab ( didy s552 ) zebrafish embryos were a kind gift from Herwig Baier. Adult HuC:GFP zebrafish were a kind gift from Stephen Ekker. Zebrafish were generated and maintained in accordance with the guidelines of the University of California, San Francisco, Committee on the Use and Care of Animals. Zebrafish larvae were maintained in ‘embryo medium’ consisting of 0.03% Instant Ocean (Aquarium Systems, Inc., Mentor, OH, USA) in deionized water containing 0.002% Methylene Blue as a fungicide. Larval zebrafish clutches were bred from scn1Lab heterozygous animals that had been backcrossed to Tupfel long WT or HuC:GFP zebrafish for at least seven generations. Homozygous mutants (sorted based on pigmentation) and age-matched sibling larvae were used. Although the precise genetic defect responsible for the skin pigmentation issue is unknown, it is interesting that a 1.5-fold upregulation of a gene encoding the melanocortin 5a receptor was noted in our microarray data. Seizure monitoring Procedures for locomotion tracking and electrophysiology were described [24] , [27] . In pilot experiments, HuC:GFP zebrafish were used in electrophysiology experiments to obtain an estimation of the location of recording electrodes. Locomotion plots were obtained for one fish per well at a recording epoch of 10 min using a DanioVision system running EthoVision XT software (Noldus Information Technology, Leesburg, VA, USA). Seizure scoring was performed as described [27] . Locomotion plots were analysed for distance travelled (in mm) and mean velocity (in mm s −1 ). Epileptiform events were analysed in pClamp (Molecular Devices, Sunnyvale, CA, USA) and defined as upward or downward membrane deflections greater than 2 × baseline noise level, and were classified as interictal-like (100 to 300 ms duration) or ictal-like (1,000 to 5,000 ms duration). Burst frequency was determined by counting the number of epileptiform events per minute during a 10-min recording epoch. Burst duration was determined by measuring the onset-to-offset interval for all events during the same epoch. Drugs Drugs were obtained from Sigma-Aldrich and were dissolved in embryo media. Stock solutions were prepared in embryo media at 1 mM and pH adjusted to ~7.5. Ganaxolone was a kind gift from BioCrea GmbH (Radebeul, Germany). Compounds for drug screening were purchased from MicroSource Discovery Systems, Inc. (International Drug Collection, Gaylordsville, CT, USA) and were provided as 10 mM dimethylsulphoxide (DMSO) solutions. Test compounds were dissolved in embryo media and tested at concentrations between 6.7 and 667 μM; final DMSO concentration ~7%. An initial screen concentration of 667 μM was chosen for behavioural studies in freely swimming fish, as this falls on the lower range of AED concentrations previously reported in to be effective against PTZ (10–20 mM)-induced seizures in larval zebrafish (0.1–25 mM) [27] , [32] , [42] and was the most efficient use of the small volume of stock solution (250 μl) provided by MicroSource Discovery Systems, Inc. A slightly higher concentration (1 mM) was chosen for the initial AED validation assays in Figs 5 and 6 to account for any potential complications associated with diffusion through the agar. DMSO was evaluated for toxicity at dilutions between 0.01 and 100% using WT larvae ( n =12 fish per concentration); DMSO at >25% was lethal. In all drug-screening studies compounds were coded and experiments were performed by investigators blind to the nature of the compound. Baseline recordings of seizure activity were obtained from mutants bathed in embryo media; a second plot was then obtained following a solution change to a test compound. Each test compound classified as a ‘positive hit’ in the locomotion assay was visually confirmed as alive based on the movement in response to touch and visible heartbeat. WT fish exhibit little to no spontaneous swim activity during these 10-min recording epochs (see Fig. 3b ) and were not used in the drug-discovery assay. Molecular biology Procedures for microarray, qPCR and whole-mount in-situ hybridization were described [25] . See Supplementary Tables S2 and S3 for primer sequence data. Data analysis Data are presented as mean and s.e.m., unless stated otherwise. Pairwise statistical significance was determined with Student’s two-tailed unpaired t -test, ANOVA or Mann–Whitney–Rank sum test, as appropriate, unless stated otherwise. Results were considered significant at P <0.05, unless otherwise indicated. How to cite this article: Baraban, S.C. et al . Drug screening in Scn1a zebrafish mutant identifies clemizole as a potential Dravet syndrome treatment. Nat. Commun. 4:2410 doi: 10.1038/ncomms3410 (2013).